Local and bulk13C hyperpolarization in nitrogen-vacancy-centred diamonds at variable fields and orientations Polarizing nuclear spins is of fundamental importance in biology, chemistry and physics. Methods for hyperpolarizing 13 C nuclei from free electrons in bulk usually demand operation at cryogenic temperatures. Room temperature approaches targeting diamonds with nitrogen-vacancy centres could alleviate this need; however, hitherto proposed strategies lack generality as they demand stringent conditions on the strength and/or alignment of the magnetic field. We report here an approach for achieving efficient electron- 13 C spin-alignment transfers, compatible with a broad range of magnetic field strengths and field orientations with respect to the diamond crystal. This versatility results from combining coherent microwave- and incoherent laser-induced transitions between selected energy states of the coupled electron–nuclear spin manifold. 13 C-detected nuclear magnetic resonance experiments demonstrate that this hyperpolarization can be transferred via first-shell or via distant 13 Cs throughout the nuclear bulk ensemble. This method opens new perspectives for applications of diamond nitrogen-vacancy centres in nuclear magnetic resonance, and in quantum information processing. Nuclear spins are central actors in nuclear magnetic resonance (NMR) spectroscopy and imaging (MRI), providing important information at the molecular, micro- and mesoscopic levels for a wide variety of physical, chemical and biological processes [1] , [2] . Owing to their long relaxation times, nuclear spins are also promising vehicles for storing and manipulating quantum information, making them useful resources for potential quantum devices that extend the limits of classical computers [3] , [4] , [5] . Many of these uses derive from the weakness of nuclear spin interactions, making NMR methods remarkably noninvasive but also the observation of NMR signals challenging and characterized by intrinsically low signal-to-noise ratios. Dynamic nuclear polarization [6] , [7] , [8] can bypass these limitations by transferring spin polarization from electrons to nuclei; for this process to be even more efficient cryogenic temperature operations are usually required [9] , [10] , [11] , leading to nuclear polarization enhancements encompassing several orders of magnitude. Electronic spins in nitrogen-vacancy (NV) centres are also promising alternatives for polarizing nuclear spins at room temperature conditions [12] , [13] , [14] , [15] , [16] , [17] , [18] , [19] . Hitherto proposed electron-to-nuclear polarization transfer methods, however, have so far demanded finely tuned energy-matching conditions, both in terms of field strength and of its orientation with respect to the diamond crystal to perform efficiently. These prerequisites pose an obstacle for utilizing these methods in generic applications, including the use of diamond powders as tracers in biological MRI injection studies [20] , [21] , [22] , or as sources to hyperpolarize nuclei outside the diamond in NMR-based analyses [23] . It is hereby shown that these demands for achieving a robust electron-to-nuclear polarization transfer can be relaxed by the inclusion of incoherent processes [24] , [25] . The method hereby proposed includes a continuous microwave (MW) irradiation that coherently addresses the 0↔−1 (or +1) S =1 electronic spin transition while exploiting the asymmetry of the electron–nucleus hyperfine (HF) interaction imposed by the spin-1 nature of the NV centre [26] , [27] , [28] , [29] . This selective MW addressing is combined with the incoherent spin repopulation effects introduced by the optical pumping process [30] , [31] to produce an imbalance between the populations of the coupled nuclear spins. This achievement of steady-state 13 C polarization is here demonstrated over a range of magnetic field strengths and orientations as well as of electron–nuclear HF interactions, both in optical studies of single NV centres and in shuttled NMR measurements of bulk samples. Moreover, by exploiting the versatility of this new approach, light is shed on the role played by HF-imposed spin–diffusion barriers in the achievement of bulk nuclear spin hyperpolarization. 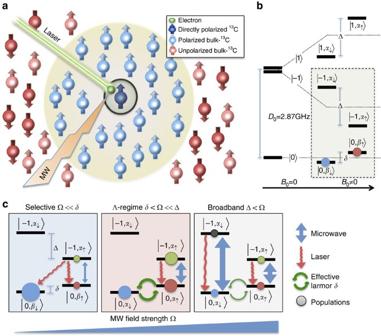Figure 1: MW-driven13C polarization derived from optically pumped nitrogen-vacancy centres. (a) Spin-1 NV electronic defect strongly coupled to a13C nucleus (black circle), irradiated simultaneously by MW (orange lightning bolt) and laser fields (green beam). The optically pumped NV-spin (green sphere) transfers its polarization to the coupled nucleus (dark blue sphere) and eventually to the remaining13C (the bulk) by interactions within a dipolar spin network (light blue spheres). The red spheres are unpolarized nuclei. (b) Energy-level diagram of the electron defect, hyperfine coupled to a13C in presence of a potential magnetic fieldB0(without MW fields). The dashed box shows the energy levels addressed, and stresses an initial state containing equal populations on the lower,eigenstates after optical pumping. (c) Spin dynamical regimes determined by the relation between the MW power and the energy splittings. The solid black lines only represent the eigenstates,,andof the system in the selective regime; in the remaining cases these lines represent states,,andthat are relevant for the MW selection rules, but whereandare linear superpositions of the eigenstatesand. Blue vertical arrows represent the MW excitation on resonance with the transition, circular green arrows represent an effective Larmor precession with frequencyδ, while curly red arrows represent a laser-induced relaxation-like process conserving the nuclear spin state but driving the incoherentoptical pumping52. The filled and coloured circles schematize the populations of each state resulting from these dynamics. Although not explicitly shown in these energy-level diagrams, the electronic and nuclear spins involved in these manifolds are also coupled by dipole–dipole interactions to the13C ensemble via a spin-coupling network, enabling further polarization transfers to the bulk (a). The MW-driven-relaxation-aided polarization transfer scheme Figure 1a defines the relevant system and active interactions that will be used to introduce our polarization transfer proposal. The system involves a single NV S =1 spin exhibiting a ground-state zero-field splitting D 0 =2.87 GHz. This electronic spin is coupled to nearby or distant 13 C nuclear spins ( I =1/2) through HF interactions and can be optically pumped to populate the electronic m s =0 level [30] , [31] . The application of a weak static magnetic field induces an additional splitting of the electronic/nuclear states, leading to the energy-level diagram in Fig. 1b . Our scenario assumes a selective MW irradiation that solely addresses the electron spin transitions, allowing one to treat the system as a four-level manifold ( Fig. 1b ). The nuclear spin components of the eigenstates associated with m s =0 ( and ) and m s =−1 ( and ) have different quantization axes because of the asymmetry imposed by a HF interaction that is absent if the electron state is m s =0 and present if m s =−1 (refs 26 , 27 , 28 , 29 ). As further discussed in Methods and Supplementary Note 1 , the corresponding eigenenergies exhibit splittings δ and Δ for the 0 and −1 manifolds, respectively. Notice that this asymmetry is due to the S =1 nature of the NV centre, and not due to particular details of couplings within the sample. These differences in level splitting and in quantization axes among nuclear spins that are initially unpolarized are here exploited to hyperpolarize them. Figure 1: MW-driven 13 C polarization derived from optically pumped nitrogen-vacancy centres. ( a ) Spin-1 NV electronic defect strongly coupled to a 13 C nucleus (black circle), irradiated simultaneously by MW (orange lightning bolt) and laser fields (green beam). The optically pumped NV-spin (green sphere) transfers its polarization to the coupled nucleus (dark blue sphere) and eventually to the remaining 13 C (the bulk) by interactions within a dipolar spin network (light blue spheres). The red spheres are unpolarized nuclei. ( b ) Energy-level diagram of the electron defect, hyperfine coupled to a 13 C in presence of a potential magnetic field B 0 (without MW fields). The dashed box shows the energy levels addressed, and stresses an initial state containing equal populations on the lower , eigenstates after optical pumping. ( c ) Spin dynamical regimes determined by the relation between the MW power and the energy splittings. The solid black lines only represent the eigenstates , , and of the system in the selective regime; in the remaining cases these lines represent states , , and that are relevant for the MW selection rules, but where and are linear superpositions of the eigenstates and . Blue vertical arrows represent the MW excitation on resonance with the transition , circular green arrows represent an effective Larmor precession with frequency δ , while curly red arrows represent a laser-induced relaxation-like process conserving the nuclear spin state but driving the incoherent optical pumping [52] . The filled and coloured circles schematize the populations of each state resulting from these dynamics. Although not explicitly shown in these energy-level diagrams, the electronic and nuclear spins involved in these manifolds are also coupled by dipole–dipole interactions to the 13 C ensemble via a spin-coupling network, enabling further polarization transfers to the bulk ( a ). Full size image Different polarization transfer routes can be activated by irradiating this HF-coupled system. We discriminate these depending on the relative MW field strength Ω vis-a-vis the energy splittings δ and Δ , determining which eigenstates will participate in the dynamics. In the selective regime ( Fig. 1c ), the MW-induced transitions involve solely two directly addressed eigenstates. Therefore, the population of a third, non-addressed state associated with the m s =0 manifold grows systematically as driven by the laser-induced relaxation processes. This generates an imbalance between the and populations, equivalent to a nuclear polarization whose direction is defined by the m s =0 eigenstate manifold. As the MW power increases, a Λ-regime where transitions are induced among three eigenstates [29] is reached ( Fig. 1c ). We describe this regime in a basis set ; here is a dark state for the MW in the sense that , and is a bright state that is addressed by the MW. Owing to the different HF properties associated with m s =0 and m s =−1, is an eigenstate but and are not, and therefore they oscillate at an effective nuclear Larmor frequency δ . As further detailed in Methods and in Supplementary Note 1 , this precession takes place around an effective field defined by the quantization axis of the states. This field is given by the nuclear Zeeman axis if the non-secular terms of the HF coupling can be disregarded; if this is not possible, a second-order perturbation approach can be used to account for the Hamiltonian determining the effective precession field (see Supplementary Figs 1–4 ). The combined action of this nuclear precession, the MW irradiation and the laser-driven relaxation results in a redistribution of the initial populations over the three-level system, biasing the bright nuclear-state population, over its dark counterpart. For the example in Fig. 1c , a net nuclear magnetization pointing along the quantization axis, defined at weak fields by the spin’s HF coupling to m s =−1, is then obtained. Finally, as the MW power is further increased, a broadband regime where the electron state is flipped without regards to the nuclear spin state is reached; in such an instance no nuclear polarization enrichment is predicted. Nuclear hyperpolarization in the vicinity of the NV centre To demonstrate these features, the local 13 C polarization achieved via this HF-mediated polarization transfer was probed by optically detected magnetic resonance experiments on a single NV centre coupled to a first-shell 13 C nuclear spin, characterized by a strong HF coupling Δ≈130 MHz (refs 26 , 29 ). 13 C polarization was measured on a crystal lattice rotated on purpose away from the external magnetic field by arbitrary Azimuthal and polar angles. The electron spin state was initialized to the m s =0 state by laser light and simultaneously irradiated with MWs for 30 μs. The eigenstate populations were then optically measured by monitoring the fluorecense emited by the NV electronic transitions, as a function of the MW frequency ω over a range covering the various transition frequencies ( Fig. 2 ; see Methods, Supplementary Notes 2–4 and Supplementary Figs 5–8 for further details). Two MW powers were used in these experiments, corresponding to the selective and Λ-regimes shown in Fig. 1 . For the selective regime, a 13 C hyperpolarization pointing along the or directions defined by the m s =0 eigenstate manifold is reached, depending on the MW irradiation frequency. For the Λ-regime, nuclear hyperpolarization is also reached but now aligned along an axis defined by the nuclear eigenstates in the m s =−1 manifold. The double-peak pattern of the eigenstate population and 13 C polarization spectra is characteristic of the selective regime. These two 13 C spin alignment maxima arise when the MW is on resonance with the transition frequencies, leading to opposite nuclear polarization directions. By contrast, in the Λ-regime, a single 13 C spin alignment peak centred between the transition frequencies is observed, evidencing that these two transitions are affected by the MW. In such a case the initial populations of the states are transferred to populate , leading to a nuclear spin alignment defined by the nuclear quantization axis. 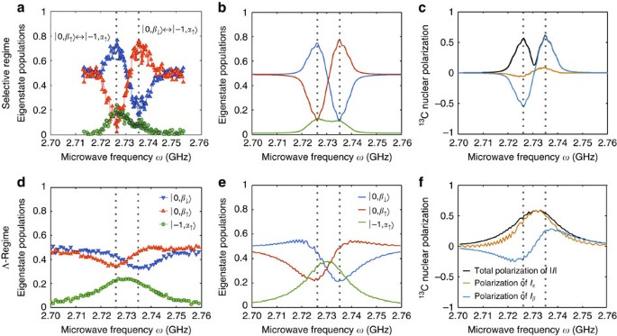Figure 2: Hyperpolarization of a first-shell nuclear spin using a MW-driven, optically pumped nitrogen-vacancy centre. Experiments were conducted by orienting a magnetic field=4.04 mT atθ≈42° andφ≈85° polar and azimuthal angles with respect to the zero-field tensorD0of the NV centre. The effective13C Larmor is thenδ≈8.8 MHz, while the first-shell hyperfine interaction is Δ≈130 MHz. Two MW power strengths were calibrated corresponding to Rabi frequencies of Ω≈1.4 MHz<8.8 MHz≈δ(a–c) and Ω≈11.9 MHz>8.8 MHz≈δ(d–f) corresponding to the selective and the Λ-regime, respectively. Blue, red and green colours represent the states,andrespectively. (a,d) Optically detected experiments determining the eigenstate populations at the end of the polarization phase during 30 μs as a function of the MW frequencyω. (b,e) Predicted eigenstate population spectra calculated without free parameters, that is, using calibrated and known couplings, and a hyperfine tensor was taken from ref.29. In the selective regime (a–c), thepopulation spectrum exhibits two peaks corresponding to thetransition frequencies, whereas in the Λ-regime (d–f) thepopulation spectrum has a single peak centred half-way between thetransition frequencies. (c,f) Derived13C polarization spectra confirming the polarization directions along the-state axis (c) and the-state axis (f) for the selective and Λ-regimes, respectively. Figure 2: Hyperpolarization of a first-shell nuclear spin using a MW-driven, optically pumped nitrogen-vacancy centre. Experiments were conducted by orienting a magnetic field =4.04 mT at θ ≈42° and φ ≈85° polar and azimuthal angles with respect to the zero-field tensor D 0 of the NV centre. The effective 13 C Larmor is then δ ≈8.8 MHz, while the first-shell hyperfine interaction is Δ≈130 MHz. Two MW power strengths were calibrated corresponding to Rabi frequencies of Ω≈1.4 MHz<8.8 MHz≈ δ ( a – c ) and Ω≈11.9 MHz>8.8 MHz≈ δ ( d – f ) corresponding to the selective and the Λ-regime, respectively. Blue, red and green colours represent the states , and respectively. ( a , d ) Optically detected experiments determining the eigenstate populations at the end of the polarization phase during 30 μs as a function of the MW frequency ω . ( b , e ) Predicted eigenstate population spectra calculated without free parameters, that is, using calibrated and known couplings, and a hyperfine tensor was taken from ref. 29 . In the selective regime ( a – c ), the population spectrum exhibits two peaks corresponding to the transition frequencies, whereas in the Λ-regime ( d – f ) the population spectrum has a single peak centred half-way between the transition frequencies. ( c , f ) Derived 13 C polarization spectra confirming the polarization directions along the -state axis ( c ) and the -state axis ( f ) for the selective and Λ-regimes, respectively. Full size image Bulk hyperpolarization at variable fields and orientations The polarized NV centre is embedded in a network of dipole–dipole-interacting nuclear spins, allowing an eventual propagation of the hyperpolarization throughout the nuclear bulk ensemble ( Fig. 1a ). Achieving an effective 13 C polarization enhancement throughout an entire diamond could have important practical NMR and MRI consequences as the source of polarization for samples in contact with the diamond, as well as for tracing purposes. Consequently, we investigated whether distant 13 C spins can benefit from the polarization transfer mechanisms observed in Fig. 2 at a local level. The bulk macroscopic 13 C magnetization was directly measured by mechanically shuttling the diamond from low fields, where MW and laser fields were applied to accomplish the electron–nuclear polarization transfer, into a 4.7-T magnet enabling bulk 13 C NMR detection ( Fig. 3a,b ). 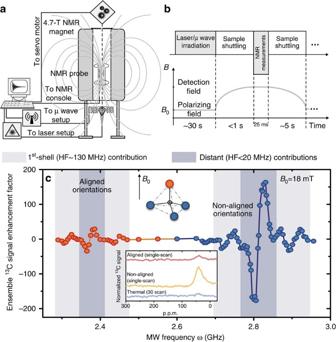Figure 3: Acquiring ensemble13C polarization spectra for varying NV orientations with respect toB0. (a) Opto-NMR set-up and (b) detection sequence used in these experiments. During the polarization transfer phase, the entire single-crystal diamond is irradiated with laser light and MW underneath the NMR magnet at a lowB0. The hyperpolarized diamond is then shuttled (in <1 s) into a 4.7-T superconducting magnet to directly detect its macroscopic13C magnetization via a spin-echo sequence. The lowB0magnetic field is aligned to one of the nitrogen-vacancy-centre orientations (in red), while the other three orientations (in blue) subtend an angle of ≈109° with respect to the field. (c) Typical13C polarization enhancement patterns observed by NMR as a function of the MW frequencyωwith signals normalized with respect to the thermal13C response at 4.7 T (inset). The left part of the plot corresponds the nuclear polarization generated byMW transitions for the aligned orientation (red circles), while the right part corresponds to nuclear polarization enhanced via the three non-aligned, equivalent orientations (blue circles). The ≈1:3 intensity ratio reflects the relative abundances of aligned and non-aligned sites in the diamond’s tetrahedral structure. In each of the patterns, the central peaks represent bulk nuclear hyperpolarization pumped via13C spins coupled with hyperfine interactions lower than 20 MHz, while the outer peaks originate from first-shell13Cs whose hyperfine splitting is ≈130 MHz (refs26,29). The antiphase structure of each of these peaks corresponds to the MW transitionsandat one side of the central peaks, and to thestate at the other side. The inset shows NMR spectra obtained for a thermally polarized sample, and at the maxima of the central peaks for the aligned and non-aligned orientations. p.p.m. refers to parts-per-million of the high-field NMR13C resonance frequency, which in our case is 50.5 MHz. Figure 3c presents results arising from a typical experiment, showing the dependence of the ensemble 13 C magnetization on the MW frequency ω . For consistency, measurements were carried out with the polarizing B 0 field aligned along one of the NV centre orientations, meaning that the remaining three orientations of the crystal form an angle of ≈109° away from the field direction. The nuclear polarization spectrum ( Fig. 3c ) shows two regions of enhancement, corresponding to the aligned and non-aligned orientations of the NV defects. Both regions show similar patterns of multiple positive and negative peaks, corresponding to different HF couplings and MW-induced transitions. Both 13 C patterns contain major central peaks, and minor outer peaks detuned by ≈±60 MHz from their centres. The central peaks correspond to bulk 13 C nuclei being hyperpolarized via 20-MHz HF interactions, that is, via 13 C spins positioned at or beyond the NV’s second shell [27] , [28] . The outer peaks also correspond to bulk 13 C polarization, but arriving this time via first-shell 13 Cs whose HF splitting is ≈130 MHz (refs 26 , 29 ). In this instance, the bulk 13 C magnetization exhibits a sign-flip pattern characteristic of the selective regime, akin to the local 13 C polarization pattern shown in Fig. 2c , although these are bulk 13 C resonances detected on the whole diamond, and not single-spin measurements. This demonstrates that 13 C ensemble hyperpolarization can be derived via either nuclear–nuclear dipole couplings involving distant spins to the electron, or via first-shell 13 C spins. The latter is a remarkable fact, given that in this case the build-up of bulk polarization needs to overcome the >60-MHz detuning characterizing the first-shell sites acting as polarization transfer bridgehead. The timescales that are then needed to achieve a bulk polarization build-up, ∼ 30 s, are orders of magnitude longer than the first-shell electron- 13 C polarization transfer time (<ms, see Supplementary Note 4 and Supplementary Fig. 7 ). This difference in timescales explains how a low-concentration, highly detuned species such as the first-shell 13 C suffices to polarize the bulk sample examined by the NMR experiments (see Supplementary Note 5 for a rough estimation of the number of polarized 13 C). 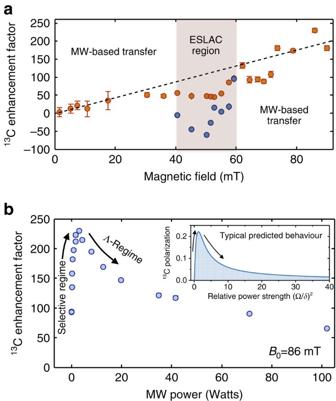Figure 4: Ensemble13C magnetization for different magnetic field strengths and MW powers. The experimental points of these panels correspond to the maximum signal of the central peak in the aligned orientation. (a)13C polarization as a function of the magnetic field strengthB0(normalized to its thermal 4.7-T counterpart and measured up to our maximum operating field, corresponding to ≈100 mT). The dashed line is a guide to the eye. Within the shaded excited-state level anticrossing (ESLAC) region polarization transfer was observed, deriving from the combined action between a level anticrossing mechanism12,13,14and the here proposed MW-induced transfer scheme. These two nuclear polarization mechanism proceeded with opposing signs. Within this region, the blue dots show the resulting signal from the combined action of the ESLAC- and MW-induced transfer, while the orange dots show the MW-induced enhancement factor after a phenomenological subtraction of the13C polarization transferred solely by the ESLAC scheme. (b)13C hyperpolarization as a function of the MW power at a fixed field of ≈86 mT. The inset shows the typical predicted behaviour by the model, where the13C polarization grows with MW power within the selective regime, but decreases as the Λ-regime is reached. As a qualitative comparison, the inset’s numerical simulations consider a single NV centre coupled to a single13C with an hyperfine interactionAzz=5Azx. In this case Δ=80δ, the laser-pumping rate=1.5/δ, the total polarization time=120/δand the MW frequency is on resonance with thetransition. Qualitatively similar behaviours are obtained for different parameters. In both panels, the error bars represent the propagated relative error of the spin signal on the calculated enhancement factors. Figure 4 further demonstrates the versatility of the method to yield bulk nuclear hyperpolarization, as evidenced by the achievement of enhanced 13 C NMR signals over a broad range of polarizing magnetic fields and of MW powers. Notice that the nuclear polarization reveals a systematic increase as a function of B 0 ( Fig. 4a ), as well as a clear optimum for the MW power ( Fig. 4b ) consistent with a transition from a selective regime in which the polarization grows with MW power to a Λ-regime in which it decreases with the MW power (see inset and Supplementary Note 4 ). Interference effects between a hyperpolarization driven by an excited-state level anticrossing [13] , [14] , [15] and the MW-induced transfer scheme introduced here are seen at fields of ∼ 50 mT. In contrast to the MW-induced transfer, the anticrossing-based technique requires that the electron/nuclear Zeeman energy detuning conditions be smaller than the dominant HF interaction. The relatively narrow range of magnetic field values compatible with this transfer scheme is thus in contrast to the MW-induced transfer processes, where matching requirements are relaxed as the MW frequency can be tuned to an array of electronic–nuclear frequency transitions (for example, Fig. 4a ). Figure 3: Acquiring ensemble 13 C polarization spectra for varying NV orientations with respect to B 0 . ( a ) Opto-NMR set-up and ( b ) detection sequence used in these experiments. During the polarization transfer phase, the entire single-crystal diamond is irradiated with laser light and MW underneath the NMR magnet at a low B 0 . The hyperpolarized diamond is then shuttled (in <1 s) into a 4.7-T superconducting magnet to directly detect its macroscopic 13 C magnetization via a spin-echo sequence. The low B 0 magnetic field is aligned to one of the nitrogen-vacancy-centre orientations (in red), while the other three orientations (in blue) subtend an angle of ≈109° with respect to the field. ( c ) Typical 13 C polarization enhancement patterns observed by NMR as a function of the MW frequency ω with signals normalized with respect to the thermal 13 C response at 4.7 T (inset). The left part of the plot corresponds the nuclear polarization generated by MW transitions for the aligned orientation (red circles), while the right part corresponds to nuclear polarization enhanced via the three non-aligned, equivalent orientations (blue circles). The ≈1:3 intensity ratio reflects the relative abundances of aligned and non-aligned sites in the diamond’s tetrahedral structure. In each of the patterns, the central peaks represent bulk nuclear hyperpolarization pumped via 13 C spins coupled with hyperfine interactions lower than 20 MHz, while the outer peaks originate from first-shell 13 Cs whose hyperfine splitting is ≈130 MHz (refs 26 , 29 ). The antiphase structure of each of these peaks corresponds to the MW transitions and at one side of the central peaks, and to the state at the other side. The inset shows NMR spectra obtained for a thermally polarized sample, and at the maxima of the central peaks for the aligned and non-aligned orientations. p.p.m. refers to parts-per-million of the high-field NMR 13 C resonance frequency, which in our case is 50.5 MHz. Full size image Figure 4: Ensemble 13 C magnetization for different magnetic field strengths and MW powers. The experimental points of these panels correspond to the maximum signal of the central peak in the aligned orientation. ( a ) 13 C polarization as a function of the magnetic field strength B 0 (normalized to its thermal 4.7-T counterpart and measured up to our maximum operating field, corresponding to ≈100 mT). The dashed line is a guide to the eye. Within the shaded excited-state level anticrossing (ESLAC) region polarization transfer was observed, deriving from the combined action between a level anticrossing mechanism [12] , [13] , [14] and the here proposed MW-induced transfer scheme. These two nuclear polarization mechanism proceeded with opposing signs. Within this region, the blue dots show the resulting signal from the combined action of the ESLAC- and MW-induced transfer, while the orange dots show the MW-induced enhancement factor after a phenomenological subtraction of the 13 C polarization transferred solely by the ESLAC scheme. ( b ) 13 C hyperpolarization as a function of the MW power at a fixed field of ≈86 mT. The inset shows the typical predicted behaviour by the model, where the 13 C polarization grows with MW power within the selective regime, but decreases as the Λ-regime is reached. As a qualitative comparison, the inset’s numerical simulations consider a single NV centre coupled to a single 13 C with an hyperfine interaction A zz =5 A zx . In this case Δ=80 δ , the laser-pumping rate=1.5/ δ , the total polarization time=120/ δ and the MW frequency is on resonance with the transition. Qualitatively similar behaviours are obtained for different parameters. In both panels, the error bars represent the propagated relative error of the spin signal on the calculated enhancement factors. Full size image A versatile method for hyperpolarizing nuclear spin ensembles at room temperature using NV centres in diamond was proposed and demonstrated. The method relies on the combined action of continuous laser light and MW irradiation, and exploits the asymmetries of the HF interaction imparted by the spin-1 nature of the NV centre. This allows us to transfer spin order from the electronic m s =0 state to the nuclei, by exploiting the evolution triggered on selectively irradiating transitions. Nuclear spin hyperpolarization is thus obtained for a broad range of magnetic field strengths and arbitrary field orientations with respect to the diamond lattice, as well as for a wide range of HF interactions. These principles may facilitate a number of applications. One entails facilitating the use of pre-polarized diamonds in NMR experiments owing to the ease with which NV electrons can be optically pumped by comparison with cryogenic-based high-field counterparts. This easing of the hyperpolarization conditions should also facilitate the use of these samples in multiscan acquisition of the kind desirable in in vivo MRI scans. Our scheme provides an approach for optically detected nanoscale NMR/MRI of polarized nuclear spin ensembles that complements methods based on spin noise thermal fluctuations [23] , [32] , [33] , [34] , [35] . The fact that the method works for different orientation and strengths of the magnetic field can be exploited for polarizing diamond powders, leading to an alternative route to NMR measurements that complements the ones based on thermal polarization. Further studies on the basis of frequency sweeps are in progress to evaluate the efficiency of the nuclear spin polarization process in powders at higher fields. Alternatively, approaching a zero magnetic field might be advantageous, since all orientations would then become nearly equivalent and addressable in a simultaneous manner. In addition to potential NMR/MRI uses, this method could be useful for dissipative nuclear-state preparation in ensemble quantum memories, for quantum information processing [36] , [37] , [38] , [39] . Hyperpolarizing nuclear spin ensembles in solid-state systems also provides a tool to study condensed matter and many-body physics phenomena of cold bodies, where quantum effects (for example, quantum phase transitions) are more sharply manifested [40] , [41] , [42] , [43] . The concepts here used might also find applicability in other kinds of cross-polarization scenarios, involving generic transfers between a spin-1 source coupled to other spins. Besides demonstrating the method’s capability at a local level, it was shown that nuclear hyperpolarization can be extended throughout the bulk ensemble by spin-diffusion—even when targeting first-shell nuclear spins strongly shifted by HF couplings. This provides a new tool for understanding the complex non-equilibrium dynamics of many-body systems, where a local polarization can be created in a controlled way and its spreading into the bulk be monitored [44] , [45] , [46] , [47] . Single-crystal sample For the single NV detection experiments the sample used was a commercially available, untreated, type IIa, electronic-grade natural abundance 13 C diamond crystal (dimension: 2 × 2 × 0.3 mm 3 ). For the NMR experiments, an isotopically enriched (10% 13 C) type Ib high-pressure, high-temperature diamond was used. The enriched crystal was grown by the temperature gradient method at a pressure of 6 GPa and a temperature of 1,700 K from Ni-2 wt% Ti solvent using a powdered mixture of 13 C-enriched and natural abundance graphic carbon. These samples were irradiated at room temperature (2 MeV, 10 h, total fluence 8 × 10 17 e cm −2 ) and annealed (2 h, 1,000 °C). Subsequent examination using confocal laser microscopy confirmed that the two most abundant paramagnetic impurities consisted of electrically neutral single substitutional nitrogen atoms (P 1 ), and charged nitrogen atoms next to a lattice vacancy forming an optically active colour centre (NV − ). The concentrations of these impurities were both <5 p.p.m. (part-per-million). In both samples, we estimate a T 1 ≈5 ms for the NV electron spin in the electronic ground state. Whereas single NV centre experiments on natural abundance 13 C samples revealed a ≈2.5 μs (ref. 48 ), for the 13 C-enriched crystal we estimate using optically detected magnetic resonance (ODMR) a ≈12 ns for the NV centre in the ground state at the polarizing fields. For the single NV centre experiments, a ≈20 μs was measured for the nuclear spin. In the 13 C-enriched diamond crystal, bulk 13 C T 1 relaxation times ranged from 5 to 20 s depending on the magnetic field strength at the polarizing fields (1–100 mT). At the detection field B 0 =4.7 T used in the 13 C bulk studies, T 1 relaxation was >10 min and =160±50 μs. System Hamiltonian At room temperature, the NV centre energy-level structure exhibits an electronic triplet as the ground state ( 3 A 2 ) [12] , [13] , [14] . The quantum Hamiltonian of a single NV defect ( S ) and one 13 C nucleus ( I ) can thus be described as . Here D 0 =2.87 GHz is the zero-field splitting term, γ e and γ n the electronic and nuclear gyromagnetic ratios, B is the magnetic field vector and A a HF tensor that depends on the specific NV and nearby 13 C spin [49] . For simplicity, we consider first a magnetic field B aligned with the axis of the zero-field tensor D 0 and the secular approximation . This Hamiltonian simplifies to , where the axis x was chosen such that A zy =0. The feature enabling the magnetization transfers illustrated in Fig. 1 is that in the m s =0 manifold the eigenstates have a nuclear component and exhibiting a nuclear Zeeman splitting δ = γ n B 0 , whereas in the m s =−1 manifold the and nuclear components of the eigenstates are quantized on a different axis determined by the HF tensor for weak magnetic fields . For the states the eigenstate splitting δ may also depend on non-secular corrections of the HF coupling, which may also lead to an effective tilt of the nuclear spin quantization away from the magnetic field B (see Supplementary Figs 1 and 2 ). By contrast, the states are not significantly modified by the non-secular HF terms if , that is, on a condition far from the level anticrossings [13] , [14] , [15] (we do not consider here the more complicated scenario when the level anticrossing conditions are fulfilled, see Supplementary Fig. 2 for further details). If the magnetic field is not aligned with the D 0 tensor, the level structure discussed in Fig. 1 remains even if the definitions of and will change [29] ; the crucial characteristic is that they will still have different quantization axes and different eigenstate splittings δ and Δ (see Supplementary Figs 3 and 4 ). For more details on the eigenstates, energy splittings and the participation of them on the polarization dynamics please refer to Supplementary Note 1 . Single NV optical set-up The single NV detection was conducted on a home-built confocal microscope. Continuous wave green laser light ( λ =532 nm) was switched by an acousto-optic modulator (Isomet, rise/fall times ≈30 ns) coupled into a single mode optical fibre and focused on the diamond sample by an oil-immersion microscope objective (Olympus, numerical aperture=1.35). The objective was placed on a three-axis piezo stage (Npoint) enabling a scan range of the x , y , z axes of 250 × 250 × 25 μm with a resolution of ∼ 1 nm. The emerging red fluorescence signal was focused into a single-photon counting module (Perkin-Elmer, dark count rate 100 counts s −1 ). To induce transitions within the ground-state triplet during the polarization and detection sequences, MW fields were produced by two copper wires attached to the diamond (diameter ∼ 50 μm). During the hyperpolarization process, the laser intensity was reduced to ∼ 5% of its saturation intensity ( P sat ∼ 1 mW at the objective’s back) to avoid light-induced nuclear-state depopulation [12] , [50] (see Supplementary Note 4 and Supplementary Fig. 8 ). Populations and polarization in single NV centre experiments The eigenstates’ populations were obtained by performing a series of complementary measurements involving selective MW irradiation on eigenstate-specific transition frequencies, followed by an optical readout of the NV centre populations (see Supplementary Note 2 and Supplementary Fig. 5 for further details). With these selective experiments and a linear system of equations, the populations of the three active eigenstates ( and ) could be reconstructed. To perform these calculations, the fluorescence levels at the end of the different polarization sequences were measured, and properly normalized by executing the schemes with and without MW irradiation ( Supplementary Fig. 6 ). In the selective regime, the MW Rabi frequency Ω =1.4 MHz was lower than the HF splitting with the 14 N nuclear spin (2.16 MHz) [51] . Therefore, to address the latter’s three nuclear spin orientations simultaneously, the MW source was further modulated to create the three corresponding frequencies spaced by 2.16 MHz (see Supplementary Note 3 ). The wiggles in Fig. 2a–c are consequence of this irradiation mechanism. The magnetic field strength and orientation were optimized to be large enough for allowing selective excitation independent of the host 14 N nuclear spin ( δ >4–5 MHz), and small enough to allow mutual excitation (that is, Λ-regime) with reasonable MW power ( δ <10 MHz). The static and MW magnetic fields and the laser-pumping rate were calibrated from ODMR spectra, and from time-resolved measurements of the Rabi oscillations and the laser-pumping evolution. The values of the static and MW fields are given in the caption to Fig. 2 , while the optical pumping rate was 1/3 μs −1 and had a pumping efficiency of ≈90%. The curves in Fig. 2b,c,e,f were obtained by solving the spins’ quantum evolution based on a quantum master equation involving the total six-level model of a single NV centre coupled to a single 13 C nuclear spin, as further detailed in Supplementary Note 2 . The bare system Hamiltonian used was introduced in the Methods section: System Hamiltonian (for further details see Supplementary Note 1 ); simulations were performed on the basis of this Hamiltonian in the rotating frame of the MW irradiation, with frequency parameters as discussed in the main text. The pumping process was modelled as a non-Hermitian relaxation process using a Lindblad form reflecting the incoherent transition from the m s =±1 states to the m s =0 state, and using the experimentally determined pumping rate 1/3 μs −1 as the relaxation rate. The HF tensor of the first-shell 13 C spin was taken from ref. 29 (see Supplementary equation (16) ). For the selective regime, the 14 N HF splitting was considered phenomenologically as an ensemble superposition of the signal coming from the three frequencies used in the MW irradiation. Set-up for the ensemble-detected nuclear spin polarization experiments In a single-crystal diamond, NV centres can be separated into subensembles corresponding to four magnetically inequivalent orientations. The diamond sample used for the optically pumped NMR measurements had a polished [100] surface orientation. The sample was rotated in B 0 until one of the NV centre orientations was aligned to the magnetic field, while the three remaining subensembles were degenerate at an angle of ∼ 109° forming the non-aligned orientations. The weak magnetic field in these experiments ( B 0 =0–100 mT) was provided by the stray field of the superconducting magnet used to perform the bulk high-field NMR measurements, connected by a compensating low-field coil. The laser light was produced by a diode-pumped solid-state laser (Verdi-V10, λ =532 nm) coupled into an optic fibre and then focused to either partially or fully illuminate the diamond crystals. To avoid excessive heating during the optical pumping, the sample was immersed into a transparent water-filled flask and vented with pressurized air to keep the temperature constant. For the application of continuous wave MW irradiation, radio- and MW signals from a broadband frequency synthesizer were amplified by up to +30 dB for frequencies ω >600 MHz and up to +43 dB for ω <600 MHz. These amplified signals were then fed into a Helmholtz coil electronic circuit tuned to 50 Ω. The bulk 13 C experiments began with a combined laser and MW irradiation (10–30 s) to optically initialize the electronic spins and induce a transfer of the ensuing hyperpolarization from the electronic to the nuclear spins. The sample was then rapidly (<0.5 s) shuttled from the polarizing field B 0 to the sweet spot of the high-field (4.7 T) NMR magnet, where the nuclear spins were subject to a pulsed detection using an NMR probe with a Helmholtz coil configuration tuned to 50.55 MHz. The observed NMR signal consists of a single optically enhanced 13 C spectral line resonating at ca. 60 p.p.m. with a linewidth between 1 (natural abundance) and 3 kHz (10% enriched crystal). The sample then returned to the polarizing field for a repeated cycle of optical pumping and MW irradiation for the purpose of signal averaging. How to cite this article: Álvarez, G. A. et al. Local and bulk 13 C hyperpolarization innitrogen-vacancy-centred diamonds at variable fields and orientations. Nat. Commun. 6:8456 doi: 10.1038/ncomms9456 (2015).